Multicolor ultralong phosphorescence from perovskite-like octahedral α-AlF3 Designing organic fluorescent and phosphorescent materials based on various core fluorophore has gained great attention, but it is unclear whether similar luminescent units exist for inorganic materials. Inspired by the BX 6 octahedral structure of luminescent metal halide perovskites (MHP), here we propose that the BX 6 octahedron may be a core structure for luminescent inorganic materials. In this regard, excitation-dependent color-tunable phosphorescence is discovered from α-AlF 3 featuring AlF 6 octahedron. Through further exploration of the BX 6 unit by altering the dimension and changing the center metal (B) and ligand (X), luminescence from KAlF 4 , (NH 4 ) 3 AlF 6 , AlCl 3 , Al(OH) 3 , Ga 2 O 3 , InCl 3 , and CdCl 2 are also discovered. The phosphorescence of α-AlF 3 can be ascribed to clusterization-triggered emission, i.e., weak through space interaction of the n electrons of F atoms bring close proximity in the AlF 6 octahedra (inter/intra). These discoveries will deepen the understanding and contribute to further development of BX 6 octahedron-based luminescent materials. Luminescent materials are indispensable for our daily life, especially in lighting, displaying, and imaging-related applications [1] , [2] . Therefore, luminescent materials design (either organic or inorganic) is of great importance and attracts great attention. It is widely accepted that luminescence from organic materials can be ascribed to their core structure in most cases (Fig. 1 , together with the substituents), for example, fluorescent materials from xanthene [3] , [4] , [5] , [6] , [7] and phosphorescent materials based on carbazole [8] , [9] , [10] , [11] . Such core structure endow organic fluorophores with great flexibility and processability. While for inorganic luminescent materials, although structurally diverse and mostly acting as host materials for doping of transition- or rare-earth metal ions (e.g., ZnS [12] and SrAl 2 O 4 [13] ), core structure as the light-emitting unit has seldom been reported and explored like organics. So, is there similar core structure for the luminescent inorganic materials? Fig. 1: Schematic illustration of luminescent materials design. Inspired by the general luminescent material design based on organic core fluorophores and the widely investigated metal halide perovskites, here, we proposed BX 6 octahedral unit as inorganic luminescent core structure. Full size image All-inorganic metal halide perovskites (MHPs), a type of semiconductor materials with excellent photoelectric properties [14] , have been widely used in solar cells [15] , LED [16] , and thermoelectric modules [17] . The core structure of luminescent MHPs can be described as the BX 6 octahedron (Fig. 1 ), which is constituted by the central cation (B, hexa-coordinated) and six halide ligands (X=Cl, Br, I). Normally, the BX 6 octahedron is organized in an all-corner-sharing 3D network. Due to the adjustable octahedral connectivity, a series of lower dimensional metal halide-based luminescent perovskite derivatives have been reported [18] . On the other hand, the central cation and ligand halides could be altered, leading to tunable luminescence performance from 3D and lower dimension metal halides [19] , [20] . Therefore, the BX 6 octahedron is an important structure for the luminescence of MHPs, but whether such unit can be generalized for other luminescent inorganic materials remains unexplored. In this work, we find that inorganic materials constructed by the BX 6 octahedron exhibit interesting long-lived room temperature phosphorescence (RTP), i.e., the BX 6 octahedron may be regarded as a basic unit for the luminescent inorganic materials. For example, α-AlF 3 , the material constructed by AlF 6 (the lightest BX 6 octahedron) with 3D perovskite-like structure [21] , shows color-tunable RTP (up to 7 s for the blue emission). When lowering the dimension of the AlF 6 octahedron, luminescence from KAlF 4 (2D) and (NH 4 ) 3 AlF 6 (0D) is also discovered. Moreover, by changing B and X in the octahedral emissive unit of BX 6 , luminescence from AlCl 3 , Al(OH) 3 , Ga 2 O 3 , InCl 3 , and CdCl 2 are also obtained. Similar to BX 6 octahedron-based MHPs, the luminescence from AlF 3 exhibit typical self-trapped exciton (STE) emission. Besides, the octahedron also brings close proximity of F atoms, resulting in weak through-space interaction of the n electrons in F atoms for clusterization-triggered emission (CTE, recently found in n electron-rich organics for excitation-dependent color-tunable phosphorescence [22] , [23] , [24] ). 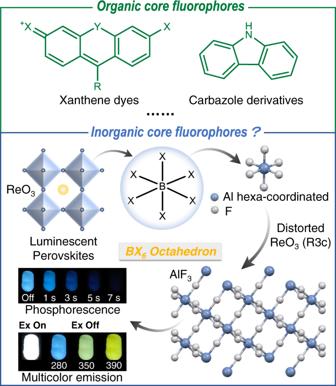Fig. 1: Schematic illustration of luminescent materials design. Inspired by the general luminescent material design based on organic core fluorophores and the widely investigated metal halide perovskites, here, we proposed BX6octahedral unit as inorganic luminescent core structure. It should be noted that it is normally the heavy atoms that drives the formation of triplet and phosphorescence in inorganics (e.g., previous Al-based luminescent materials, Supplementary Table 1 ). However, α-AlF 3 contains only light elements. Therefore, the discovery here is interesting for both organic and inorganic phosphors. In addition, the intriguing color-tunable phosphorescence without extra sophisticated molecular design can be explored for facile UV light detection with visible colored afterglow emission as readout. Luminescence of α-AlF 3 To investigate the luminescent properties of the BX 6 octahedron, hexa-coordinated AlF 6 was chosen first. Considering its outermost electronic structure (3 s 2 3 p 1 ), aluminum is lightest atom to generate the octahedral structure. Meanwhile, F ‒ is the smallest anion [25] that can coordinate with Al 3+ . The corner shared octahedra of AlF 6 results in the formation of three-dimensional network of α-AlF 3 (Fig. 1 ). Normally, AlF 3 is used as the electrolyte regulator in the aluminum smelting industry for increasing the melting point and conductivity. 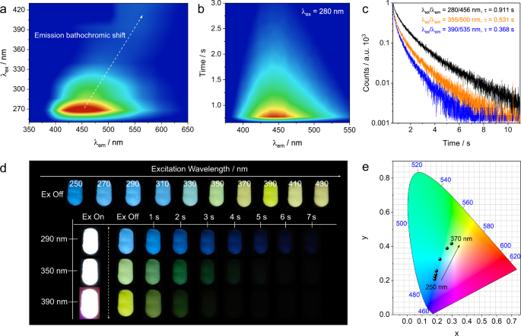Fig. 2: Luminescence properties of α-AlF3(calcinated from AlF3·3H2O). aexcitation- phosphorescence emission mapping of AlF3(delay time: 40 ms);btime-resolved emission spectra (TRES, λex= 280 nm) of AlF3;clifetime decay profiles of phosphorescent emission excited at 280, 355, and 390 nm, respectively;dphotographs taken under different excitation (250 to 430 nm) off and afterglow emission images excited at 290, 350 and 390 nm, respectively (the excitation-dependent afterglow can be observed in the excitation range from 250 to 510 nm at room temperature condition);eCIE coordinates of AlF3phosphorescence under different excitation (250 to 370 nm). 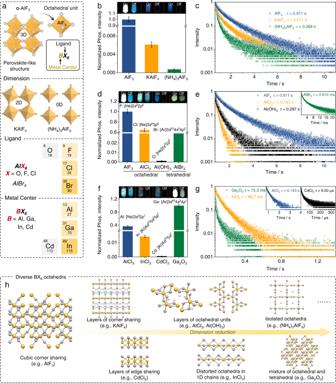Fig. 3: Investigation on the BX6octahedral luminescent unit. a, schematic diagram of chemical structure of AlF3and engineering of the octahedral basic unit;bandc, relative phosphorescence intensity and lifetime decay profiles (λex= 280 nm) of the phosphorescence emission at 456, 480, 446 nm of AlF3, KAlF4, and (NH4)3AlF6, respectively;d,e, relative phosphorescence intensity and lifetime decay profiles (λex= 280 nm) of the phosphorescence emission at 456, 486, 450, 496 nm of AlF3, AlCl3, Al(OH)3, and AlBr3, respectively;f,g, relative phosphorescence intensity, and lifetime decay profiles (λex= 280 nm) of the phosphorescence emission at 486, 468, 460, 500 nm of AlCl3, InCl3, CdCl2, and Ga2O3, respectively; andh, summary of the diverse crystalline structures of the luminescent comprising BX6octahedra. Error bars represent standard deviation (n= 3). However, its photophysical properties are rarely studied. Here, we found AlF 3 exhibited exciting color-tunable luminescence at room temperature (Fig. 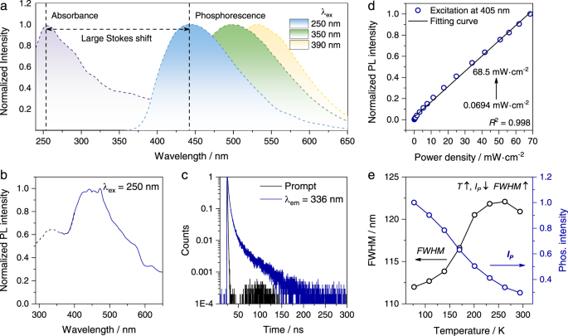Fig. 4: Investigation of the STE emission of AlF3. aAbsorbance and phosphorescence spectra (λex= 280, 350, and 390 nm, respectively.);bNormalized PL spectra (λex= 250 nm, the dotted line was measured without long pass filters, while the dashed line with 341 nm long pass filter placed at the emission exit);clifetime of AlF3monitored at 336 nm (λex= 280 nm);dplot of PL intensity as a function of excitation power density (λex= 405 nm);eplots of FWHM and intensity of phosphorescence as a function of temperature (λex= 280 nm; delay time: 40 ms). 2a and Supplementary Fig. 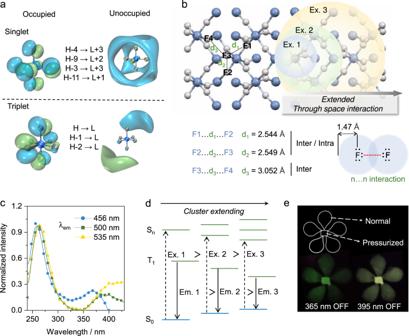Fig. 5: Investigation of the phosphorescence of AlF3. athe TD-DFT calculated isosurfaces of occupied and unoccupied orbitals of excited singlet state with maximum oscillator strength and lowest triplet excited state in AlF6octahedral unit.bstructural analysis of α-AlF3(crystalline structure from ISCD 68826).cexcitation spectra (λem= 456, 500, and 535 nm, respectively.) of α-AlF3dschematic energy level diagram of AlF3from one octahedron to network.ePhotograph of AlF3afterglow with a flower pattern, consisting of untreated and pressure-treated α-AlF3, respectively. 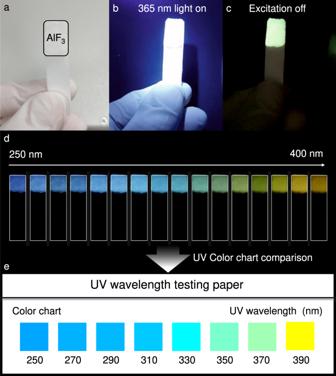Fig. 6: UV wavelength detection with AlF3-loaded testing paper. aillustration of the testing paper coated with AlF3;ba beam of UV excitation irradiated on the testing paper;cAlF3-testing paper phosphorescence demonstration after ceasing 365 nm excitation;dmulticolor phosphorescence from the AlF3-tesing paper after ceasing a series of UV excitation;ecolor chart of UV wavelength testing paper. 3 ), irrespective of its origins (Supplementary Table 6 and Fig. 2 ). From the time-resolved emission spectra (TRES, Fig. 2b and Supplementary Fig. 11 ), the luminescence of α-AlF 3 could be attributed to phosphorescence, with quantum yield (Φ P ) of ~4.22% and lifetime up to ~0.9 s (λ ex = 280 nm, Fig. 2c ). The room-temperature afterglow of α-AlF 3 could last more than 7 s (naked eye observable), and the excitation-dependent blue to yellow afterglow could be visualized clearly after ceasing the excitation (Fig. 2d , Supplementary Figs. 12 – 13 , and Supplementary Movies 1 – 3 ). The color-tunable emission was also clearly revealed by the Commission Internationale de l’Eclairage (CIE) chromaticity coordinates (Fig. 2e ). In addition, pure white light emission could be obtained (approaching CIE of 0.33, 0.33) when changing λ ex from 270 nm to 390 nm (Fig. 2d and Supplementary Fig. 15 ). Fig. 2: Luminescence properties of α-AlF 3 (calcinated from AlF 3 ·3H 2 O). a excitation- phosphorescence emission mapping of AlF 3 (delay time: 40 ms); b time-resolved emission spectra (TRES, λ ex = 280 nm) of AlF 3 ; c lifetime decay profiles of phosphorescent emission excited at 280, 355, and 390 nm, respectively; d photographs taken under different excitation (250 to 430 nm) off and afterglow emission images excited at 290, 350 and 390 nm, respectively (the excitation-dependent afterglow can be observed in the excitation range from 250 to 510 nm at room temperature condition); e CIE coordinates of AlF 3 phosphorescence under different excitation (250 to 370 nm). Full size image To exclude the potential influence from trace impurities, direct synthesis of AlF 3 through exposing aluminum metal of the highest purity available to HF vapor was carried out. As expected, similar emission properties were also obtained (Supplementary Figs. 6 - 7 ), confirming that the luminescence was exactly from AlF 3 . Furthermore, the purchased and as-prepared samples were processed by calcination, ball milling, and acid-washing, and no appreciable change of the luminescence property was received (Supplementary Figs. 8 - 10 ). Extending of the BX 6 octahedral luminescent unit Since the 3D perovskite-like structure of α-AlF 3 is constituted by the AlF 6 octahedron, the basic unit of BX 6 was further explored by adjusting the dimension of the octahedra (Fig. 3a ). As shown in Figs. 3 b and 3c , phosphorescence from KAlF 4 (2D, layers of corner-sharing AlF 6 octahedra and BCC coordinated K + ) and (NH 4 ) 3 AlF 6 (0D, isolated AlF 6 octahedra surrounded by NH 3 ligands) was also collected (Supplementary Figs. 22 and 25 ), accompanied with similar excitation-dependent emission. 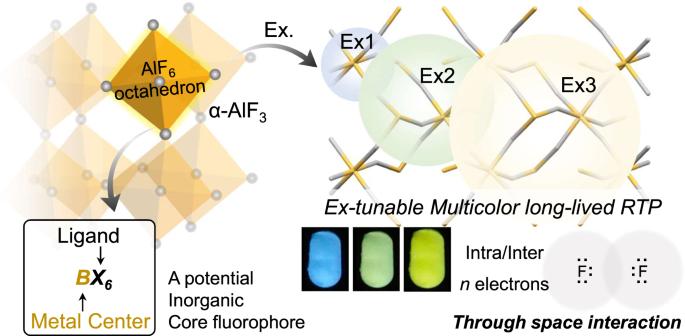Fig. 7: Summary on the BX6octahedra-based luminescence. Here, the luminescence mechanism of perovskite-like α-AlF3(and also others) was ascribed to clusterization-triggered emission ofnelectron-rich AlF6octahedrons, thus exhibiting excitation-tunable multicolor long-lived RTP. The crystalline structure information (Supplementary Table 7 ) and XRD patterns confirmed that both KAlF 4 and (NH 4 ) 3 AlF 6 were composed by the AlF 6 octahedral unit and belonged to 2D and 0D metal halides structures (Supplementary Fig. 20 ), respectively. It should be noted that lowering the dimension of the octahedra resulted in largely decreased phosphorescence intensity and shortened lifetime (Fig. 3c ), indicating that the linkage of the AlF 6 octahedra also contributed to the observed phosphorescence. Fig. 3: Investigation on the BX 6 octahedral luminescent unit. a , schematic diagram of chemical structure of AlF 3 and engineering of the octahedral basic unit; b and c , relative phosphorescence intensity and lifetime decay profiles (λ ex = 280 nm) of the phosphorescence emission at 456, 480, 446 nm of AlF 3 , KAlF 4 , and (NH 4 ) 3 AlF 6 , respectively; d , e , relative phosphorescence intensity and lifetime decay profiles (λ ex = 280 nm) of the phosphorescence emission at 456, 486, 450, 496 nm of AlF 3 , AlCl 3 , Al(OH) 3 , and AlBr 3 , respectively; f , g , relative phosphorescence intensity, and lifetime decay profiles (λ ex = 280 nm) of the phosphorescence emission at 486, 468, 460, 500 nm of AlCl 3 , InCl 3 , CdCl 2 , and Ga 2 O 3 , respectively; and h , summary of the diverse crystalline structures of the luminescent comprising BX 6 octahedra. Error bars represent standard deviation ( n = 3). Full size image Next, the ligand (X) of the BX 6 basic unit was changed with other halogens, namely AlCl 3 and AlBr 3 (Fig. 3a ). As shown in Fig. 3d and Supplementary Fig. 23 , AlCl 3 (cubic layered AlCl 6 octahedra) still exhibited appreciable long-lived phosphorescence (Fig. 3e and Supplementary Fig. 26 and Supplementary Movie 4 ). Through altering halide composition from F to Br, their emission spectra are readily tunable from blue to yellow (Insets of Fig. 3d ), which was similar with the emission tunable perovskite materials through halide engineering [26] . Although the outer space of Al is unable to accommodate six Br atoms to form stable hexadentate structure due to their relatively large atom radius discrepancy, AlBr 3 (tetrahedral) is still luminescent, but with significantly reduced intensity and shortened lifetime (Fig. 3d , 3e ). When altering the ligand from F to O, phosphorescence from the AlO 6 (octahedral) derivatives (Al(OH) 3 or Al 2 O 3 , 2D sheets of edge sharing Al(OH) 6 octahedra) was also collected (Fig. 3d and Supplementary Fig. 23 ). Upon changing the metal center of BX 6 , octahedral structure from Ga 2 O 3 (mixture of GaO 6 octahedral and GaO 4 tetrahedral), InCl 3 (distorted InCl 6 octahedra in the 1D chains), and CdCl 2 (2D sheets of edge-sharing CdCl 6 octahedra) can be expected. Again, phosphorescence from these species was successfully collected (Fig. 3f and Fig. 3g , Supplementary Figs. 23 and 27 , and Supplementary Movie 5 for Ga 2 O 3 afterglow). It should be noted that there are diverse hexa-coordinate structures evolved from different bond angles (X-B-X), thus varied phosphorescence properties (excitation, emission, intensity, and lifetime, Fig. 3h ) [27] . Luminescence mechanism of α-AlF 3 The luminescence mechanism of the octahedral unit was investigated with the 3D network AlF 6 (α-AlF 3 ). Compared with MHPs, α-AlF 3 showed the 3D perovskite-like structure, but without the insertion of alkali metal cations. These cations only contribute to lattice stabilization and does not participate in the formation of the frontier molecule orbitals [28] . The intrinsic emission of MHPs could be originated from free, bound and self-trapped excitons [29] . Among them, self-trapped exciton (STE) emission is a well-accepted mechanism to account for the broadband and large-stokes shift emission [30] , [31] , [32] , [33] . For α-AlF 3 , similar broad-band excitation-dependent blue to yellow emission was emerged, with full width at half-maximum (FWHM) of 120 nm and Stokes shift up to ~180 nm (Fig. 4a , emission spectra from λ ex = 250 nm). In addition, a high energy narrow emission at 336 nm could be identified in the broad PL spectra (Fig. 4b ), with lifetime of ~2.05 ns (Fig. 4c ). According to the previous reports [34] , [35] , such emission could be ascribed to free excitons, which can be captured by the lattice distortion due to strong electron-phonon interaction in metal halides, resulting in the generation of STE. Fig. 4: Investigation of the STE emission of AlF 3 . a Absorbance and phosphorescence spectra (λ ex = 280, 350, and 390 nm, respectively. ); b Normalized PL spectra (λ ex = 250 nm, the dotted line was measured without long pass filters, while the dashed line with 341 nm long pass filter placed at the emission exit); c lifetime of AlF 3 monitored at 336 nm (λ ex = 280 nm); d plot of PL intensity as a function of excitation power density (λ ex = 405 nm); e plots of FWHM and intensity of phosphorescence as a function of temperature (λ ex = 280 nm; delay time: 40 ms). Full size image The luminescence intensity of α-AlF 3 exhibited a linear dependence on the excitation power density (more than three orders of magnitude, Fig. 4d ), indicating that the emission is originated from photogenerated exciton (self-trapped) rather than permanent defect, the latter of which would show saturated PL intensity upon increasing the excitation power density [36] . Also, the emission band was not changed upon altering the excitation power density (Supplementary Fig. 16 ), further excluding the possibility of other emissive defects. Moreover, temperature-dependent phosphorescence spectra and cryogenic lifetime were collected (Supplementary Figs. 17 , 18 ). The emission intensity was enhanced upon lowering the temperature (294 K→77 K), accompanied by a decrease in the FWHM (Fig. 4e ), which was consistent with the characteristics of electron-lattice coupling [37] . Therefore, all these above spectral features agreed well with STE. On the other hand, although α-AlF 3 owns distorted 3D perovskite-like structure, its room-temperature phosphorescence exhibited interesting excitation-dependent feature. To further illustrate the mechanism, the transitions of AlF 3 was investigated through theoretical calculations. Considering that the BX 6 octahedra can be luminescent in isolated, corner-shared, and distorted structures, a single unit of AlF 6 was calculated with the time-dependent density functional theory (TD-DFT) [38] , [39] . The calculated excitation energy with the highest oscillator strength and the emission energy from the lowest triplet state (T 1 ) to the ground state (S 0 ) are 4.76 eV and 3.36 eV, respectively, indicating potential large Stokes shift. Next, the natural transition orbitals (NTO) were analyzed with Multiwfn [40] . As shown in Fig. 5a and Supplementary Fig. 29 , the transition with highest oscillator strength happened from the un-bonding n electron of F to the antibonding orbitals composed by the s orbital of Al and the p orbital of F. Meanwhile, such transition exhibited a typical n → σ* character, which is consistent with the deep UV absorption of AlF 3 . For phosphorescence transition (T 1 →S 0 ), the frontier orbitals comprise F 2 p (HOMO) as well as Al 3 p and F 2 p (LUMO). According to the selection rule for electronic spectra [41] , the electron transition of p - p (similar to f - f transition of lanthanides) orbitals is parity-forbidden, which is essential for the long-lived phosphorescence of AlF 3 . For the other BX 6 octahedra, similar transitions ( n → σ* ) could also be identified and their T 1 →S 0 transitions agreed well with experimental results (Supplementary Figs. 32 – 36 ). Fig. 5: Investigation of the phosphorescence of AlF 3 . a the TD-DFT calculated isosurfaces of occupied and unoccupied orbitals of excited singlet state with maximum oscillator strength and lowest triplet excited state in AlF 6 octahedral unit. b structural analysis of α-AlF 3 (crystalline structure from ISCD 68826). c excitation spectra (λ em = 456, 500, and 535 nm, respectively.) of α-AlF 3 d schematic energy level diagram of AlF 3 from one octahedron to network. e Photograph of AlF 3 afterglow with a flower pattern, consisting of untreated and pressure-treated α-AlF 3 , respectively. Full size image Recently, a number of excitation-dependent color-tunable phosphors featuring n → σ* transitions were reported, in which weak through-space interaction (TSI) was identified from the rich n electrons of the heteroatoms in the phosphors (cluster-induced emission, CIE) [22] , [23] , [24] . Structurally, α-AlF 3 is a nonconjugated system without through-bond conjugation, but F atoms with n electrons are abundant to form corner sharing networks (Fig. 5b ). Importantly, the distances between the adjacent F atoms in and between the AlF 6 octahedra (e.g., intra/inter: ~2.544 and ~2.549 Å; inter: ~3.052 Å) generally fall in the van der Waals radii of F atom (1.47 Å) [42] . Therefore, there is possible van der Waals F···F interaction, thus leading to effective electron cloud overlap of the n electrons for n → σ* transition [23] . It should be noted that F atoms also exist in NaF and KF, but no such phosphorescence could be found (Supplementary Fig. 24 ), further highlighting the importance of BX 6 octahedron. Spectrally, the excitation spectra of α-AlF 3 contains two peaks, the short wavelength of which matches with its absorption, while those at longer wavelengths red shifted upon increasing the emission wavelengths (Fig. 5c ). Besides, the excitation peaks at wavelength longer than the absorption were generally not detectable as a significant feature in the absorption spectra (Fig. 3a ), which is also a typical sign of CTE. Moreover, as further calculated with the quantum mechanics and molecular mechanics (QM/MM) method, the energy gap decreased as increasing the number of AlF 6 octahedra (increasing the sizes of the clusters, Supplementary Fig. 30 ). Therefore, different clustering states may result in varied energy gaps (Fig. 5d ), thereby excitation-dependent and color-tunable phosphorescence. The weak interaction between AlF 6 octahedra in α-AlF 3 was further investigated with Atoms in Molecules (AIM) analysis [43] . As shown in Supplementary Fig. 31 , in addition to traditional bond path in the octahedron (Al-F), there is also plenty of through-space interaction path (F···F interaction) as the AlF 6 octahedra system extended. Experimentally, upon high pressure treatment (900 MPa) to strengthen the weak intermolecular Van-der Waals interaction [44] , the emission brightness of α-AlF 3 was increased somewhat (Fig. 5e , Φ P increase from ~4.22% to ~5.46%), while the multicolor emission profiles of α-AlF 3 were not disturbed (Supplementary Fig. 19 ). Therefore, such interactions are expected to facilitate electron communications between the n electrons of F atoms and rigidify the system for efficient phosphorescence. On the basis of the above analysis, similar excitation-dependent but decreased phosphorescence intensity from KAlF 4 and (NH 4 ) 3 AlF 6 (and also other n electrons rich compounds featuring BX 6 octahedra, Fig. 3h ) can thus be expected. Lowering the dimension of the AlF 6 octahedra from 3D corner-sharing (α-AlF 3 ) to layered (KAlF 4 ) and isolated ((NH 4 ) 3 AlF 6 ) would decrease the inter-octahedra F···F interaction, thus weakening the through-space interaction (Supplementary Fig. 21 ). Moreover, the 3D corner-sharing structure may also rigidify the AlF 6 octahedra, which is beneficial for stabilization of the excited triplet states. Therefore, compared with α-AlF 3 , lowering the dimension of the AlF 6 octahedra would result in sharply decreased phosphorescence intensity and lifetime in KAlF 4 and (NH 4 ) 3 AlF 6 . For other BX 6 octahedron-containing materials, different phosphorescence performances would also be expected, due to their differences in B, X, and connection of the octahedra (Fig. 3h ). RTP of α-AlF 3 for UV wavelength detection Considering that the long-lived phosphorescence from AlF 3 is color-tunable in the visible range and excitation-dependent (particularly in the UV range), it was simply and conveniently explored for ultraviolet wavelength detection in a testing paper manner. As demonstrated in Fig. 6a , after mixed with Aloe vera gel for fixing, AlF 3 was coated on the filter paper. Upon UV irradiation, white luminescence from AlF 3 was excited (Fig. 6b ). After ceasing of UV excitation, visible afterglow images could be obtained (Fig. 6c and Supplementary Movie 6 ). Notably, upon excited with UV light of different wavelengths, the afterglow emission varied from blue to orange, which could be further compared with standard color chart to confirm UV excitation wavelength (Fig. 6d and Fig. 6e ). Such application provided a method for unknown UV wavelength detection and offered rapid and simple standard screening and testing of commercially UVA and UVB ultraviolet lamps available. Fig. 6: UV wavelength detection with AlF 3 -loaded testing paper. a illustration of the testing paper coated with AlF 3 ; b a beam of UV excitation irradiated on the testing paper; c AlF 3 -testing paper phosphorescence demonstration after ceasing 365 nm excitation; d multicolor phosphorescence from the AlF 3 -tesing paper after ceasing a series of UV excitation; e color chart of UV wavelength testing paper. Full size image In this work, perovskite-like octahedral BX 6 was proposed a basic unit for luminescent inorganic materials. In this regard, we found that α-AlF 3 (constituted by vertex sharing AlF 6 octahedral unit) exhibited long-lived color-tunable phosphorescence emission, which could last up to 7 s and be observed by naked eyes. Besides, by lowering the dimension of the AlF 6 octahedron and changing B and X in the BX 6 octahedron, luminescence from KAlF 4 , (NH 4 ) 3 AlF 6 , AlCl 3 , Al(OH) 3 , Ga 2 O 3 , InCl 3 , and CdCl 2 were also obtained. The phosphorescence of AlF 3 could also be explained with the well-accepted STE mechanism of perovskite BX 6 octahedra, together with the clusterization-triggered emission of n electron-rich phosphors. Therefore, BX 6 octahedron may be a universal structure motif for inorganic luminescent materials (Fig. 7 ). Fig. 7: Summary on the BX 6 octahedra-based luminescence. Here, the luminescence mechanism of perovskite-like α-AlF 3 (and also others) was ascribed to clusterization-triggered emission of n electron-rich AlF 6 octahedrons, thus exhibiting excitation-tunable multicolor long-lived RTP. Full size image For a long time, it has been well-accepted that there are core structures for organic luminescent materials, and their general photophysical properties can thus be interpreted. For inorganic luminescent materials, such core structure remains elusive. Our results here indicated that the boundary between the above two may be somewhat vague. Inorganic AlF 3 (also AlCl 3 , Ga 2 O 3 , and etc. ), featured with perovskite-like octahedral BX 6 basic unit, can emit long-lived phosphorescence very much similar to CTE from non-conjugated organic luminophores [22] . Moreover, typical n → σ* transition was found in the single unit of AlF 6 , which is also the typical character of CTE. Therefore, future development of luminescent materials integrating of both organic and inorganic luminescence mechanisms is expected to be appealing, particularly in MOFs containing both inorganic and organic units. Last, in the long history of the afterglow phosphor family, the IIIA group elements contributed heavily (Supplementary Table 1 , 2 ), particularly Al- and Ga-containing materials (e.g., the well-known SrAl 2 O 4 :Eu 2+ -Dy 3+13 and ZnGa 2 O 4 :Cr 3+ [45] ). However, the luminescence center are mostly lanthanides or transition metal ions [46] (e.g., Mn 2+ , and Cr 3+ ). Here, Al- and Ga-containing afterglow phosphors with ~4% QY (e.g., AlF 3 and Ga 2 O 3 ) are discovered. Particularly, the luminescence is come from the Al- and Ga-involved octahedral unit, not the dopants. Therefore, there is still much room for the exciting IIIA group chemistry in luminescent materials design. Preparation of AlF 3 AlF 3 was prepared through calcination of AlF 3 ·3H 2 O (99.9%, Macklin) at 350 °C for 3 h. To eliminate potential organic impurities, other AlF 3 samples were also subjected to the same calcination process as above. In addition, direct synthesis of AlF 3 was carried out through exposing aluminum metal (Aladdin, 99.999%, the highest purity available) to HF vapor from hydrofluoric acid (Macklin, 49wt. % in H 2 O, 99.99998%) for 3 h, followed by calcination at 350 °C for 3 h. Phosphorescence measurements Phosphorescence spectra were collected on HORIBA FluoroMax-4P with a delay time of 40 ms. For the temperature-dependent emission spectra, a model Optistat CF2 liquid nitrogen chamber (Oxford Instruments) was used and coupled with the FluoroMax-4P spectrofluorometer. Phosphorescence lifetime and the time-resolved emission spectra (TRES) were collected on HORIBA FluoroLog-3 spectrofluorometer with 280, 355, and 390 nm spectraLED as the excitation sources, respectively. The absorption spectra of solid sample were measured on Shimadzu UV-3600 with an integrating sphere unit. The phosphorescence quantum yield (Ф p ) of samples were measured in an integrating sphere (IS80, Labsphere) using 2-fluorophenylboronic acid (Ф p = 0.98% [47] ) as the reference 48 . Afterglow images The samples were excited with light selected from the Xe lamp in the Fluolog-3 spectrofluorometer (250 to 510 nm) [48] . The shutting of the excitation was controlled by instrumental software. The camera started to record video for 10 s after the excitation was turned off immediately. Theoretical calculation Theoretical calculations for the octahedral unit were performed on Orca program package (Revision 4.1.1). The ground states (S 0 ) were fully optimized by M062X with ma-def2-TZVP basis set. The excitation energies in the n-th singlet (S n ) and n-th triplet (T n ) states were obtained using the time-dependent density functional theory (TD-DFT) method based on an optimized molecular structure. In order to explore detailed excited state properties, NTO (Natural transition orbitals) analysis and hole-electron analysis method were further employed using Multiwfn program. For different cluster sizes of the AlF 6 octahedra, QM/MM method was applied to obtain optimized structure of isolated, layered and cubic corner sharing AlF 6 octahedra performed in the Gaussian 09 package [49] . The central AlF 6 octahedra were treated at the (TD) M062X/6-31G+ (d,p) level, while the surrounding molecules were treated with universal force field (UFF). For the weak interaction between AlF 6 octahedra, AIM analysis was carried out, which dictates the form of atoms in molecules and analyzes the topology of electron density. Typically, the results could be characterized by “critical points” of, namely bond (BCP), ring (RCP) and cage (CCP) critical points, representing the extreme points of electron density on the bond paths, centers of rings, and enclosed space formed by rings, respectively. It was further employed using Multiwfn program. The molecular orbitals (MO) and AIM models were all displayed using VMD. UV wavelength testing paper α-AlF 3 was mixed with Aloe vera gel with mass ratio of ~1: 1, followed by fixing on the filter paper to make the mixture evenly distributed and drying. For UV wavelength detection, the testing paper was first subjected to UV excitation for 5 seconds, then the afterglow images were either naked eye observed or photo taken with a camera.